Adaptive self-assembly and induced-fit transformations of anion-binding metal-organic macrocycles Container-molecules are attractive to chemists due to their unique structural characteristics comparable to enzymes and receptors in nature. We report here a family of artificial self-assembled macrocyclic containers that feature induced-fit transformations in response to different anionic guests. Five metal-organic macrocycles with empirical formula of M n L 2 n (M=Metal; L=Ligand; n =3, 4, 5, 6, 7) are selectively obtained starting from one simple benzimidazole-based ligand and square-planar palladium(II) ions, either by direct anion-adaptive self-assembly or induced-fit transformations. Hydrogen-bonding interactions between the inner surface of the macrocycles and the anionic guests dictate the shape and size of the product. A comprehensive induced-fit transformation map across all the M n L 2 n species is drawn, with a representative reconstitution process from Pd 7 L 14 to Pd 3 L 6 traced in detail, revealing a gradual ring-shrinking mechanism. We envisage that these macrocyclic molecules with adjustable well-defined hydrogen-bonding pockets will find wide applications in molecular sensing or catalysis. Coordination-driven self-assembly has become one of the most convenient strategies for the bottom-up construction of functional molecular ensembles [1] , [2] , [3] , [4] , [5] . On the basis of elaborate symmetry considerations, numerous two-dimensional (2D) and three-dimensional (3D) architectures have been obtained in ease by the simple combination of designed ligands (L) and metal ions (M), which show great potential in the modulation of reactivity and/or photoelectric properties of guest molecules by encapsulation [6] , [7] , [8] , [9] , [10] . To ensure the directed assembly, rigid ligands are most often employed [5] , [11] , [12] . Flexible ligands, which usually give rise to interconvertible architectures, are far less utilized in coordination-directed self-assembly [13] . However, assemblies available in nature favour flexibility over rigidity. For example, enzymes are rather flexible structures, the active site of which is continuously reshaped by interactions with specific substrates, following the so called induced-fit mechanism [14] . Anion receptor chemistry has witnessed great advances in the past decades. This area of supramolecular chemistry has a number of potential applications in biology, environment and the food industry [15] , [16] , [17] . The fast developing coordination-driven supramolecular chemistry has provided enormous examples of metal-organic assembled systems that can recognize, respond to, or sense negative-charged species [18] , [19] , [20] , [21] , [22] . However, most metal-organic receptors reported so far are of invariant structures, aiming to reach high selectivity towards targeting anions. Adaptive anion receptors, that is, receptors that can continuously transform its shape and size to maximize the binding interactions with different anions, remain elusive [23] , [24] , [25] , [26] . For example, seminal work by Hasenknopf et al . [23] has shown that use of flexible tris-bipy ligands and iron(II) lead to the formation of a dynamic combinatorial system [27] , [28] , [29] , where a set of circular helicates is expressed depending on the anions present during the self-assembly process. Herein, we report an artificial assembly system that features adaptive self-assembly and induced-fit transformation properties in the presence of anionic guests. A family of metal-organic macrocycles with the general formula of Pd n L 2 n ( n =3, 4, 5, 6, 7) are selectively obtained starting from one simple ligand and square-planar Pd II ions. Hydrogen bonding between the inner surface of the macrocycles and the bound guests, different anions in this case, dictates the shape and size of the final product. In situ anion-adaptive self-assembly gives rise to the Pd n L 2 n species for n =3, 6, 7. For n =4, 5, post-synthetic transformations [26] , [30] , [31] , [32] , [33] , [34] from other macrocycles are employed, featuring an induced-fit transformation process. Five distinct macrocycles are clearly characterized by NMR, ESI-TOF-MS, and in the case of n =3, 4, 5, 6 by single crystal X-ray diffraction. Moreover, a comprehensive map showing all the transformations across the macrocyclic species was drawn, with a representative reconstitution process from Pd 7 L 14 to Pd 3 L 6 traced in detail by titration experiments, revealing a gradual ring-shrinking mechanism. Syntheses and characterization of metal-organic macrocycles 2–6 It is well-established that self-assembly of rigid planer bidentate pyridinyl ligands with specific bent angles and square-planar Pd II ions will lead to a group of Pd n L 2 n molecular spheres [35] , [36] , [37] , [38] , [39] , [40] , [41] , [42] . Considering the inherent topological relationships, we propose that macrocyclic complexes may also be obtained when the ligand is nonplanar [43] . In this study, we choose a very simple nonplanar bidentate ligand ( 1 ) and Pd II ions as our building blocks ( Fig. 1 ). Ligand 1 has two unique features: first it is not conjugated, so that two benzoimidazole rings are reasonably free to rotate and bent, giving rise to the conformational flexibility of its coordination geometry [44] ; and second benzoimidazole bears an acidic CH bond that can act as hydrogen-bond donor, especially after its coordination to a metal [45] , [46] . In fact, varieties of anion-binding hosts utilizing the imidazole motif, either of pure organic or metal-organic forms, have been reported [47] . We envisage that anions with different size and shape will dictate the arrangement of ligand 1 during the self-assembly process, thus providing the driving force for the otherwise complicated system towards thermodynamically preferable outcome. 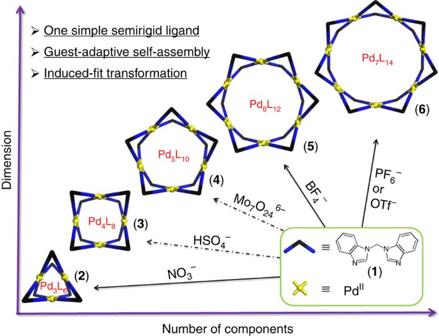Figure 1: Self-assembly of anion-binding metal-organic macrocycles. Self-assembly of anion-binding metalorganic macrocycles with an empirical formula of PdnL2n(n= 3, 4, 5, 6, 7). Dashed arrows indicate that Pd4L8and Pd5L10were obtained by induced-fit transformation from other macrocycles instead of direct self-assembly. Figure 1: Self-assembly of anion-binding metal-organic macrocycles. Self-assembly of anion-binding metalorganic macrocycles with an empirical formula of Pd n L 2n ( n = 3, 4, 5, 6, 7). Dashed arrows indicate that Pd 4 L 8 and Pd 5 L 10 were obtained by induced-fit transformation from other macrocycles instead of direct self-assembly. Full size image Reaction of ligand 1 (20.07 μmol) with a half equivalent of Pd(NO 3 ) 2 (10.04 μmol) in 1 ml dimethyl sulfoxide ([D 6 ]DMSO) at 70 °C for 5 h leads to the quantitative formation of a single compound, as confirmed by 1 H NMR spectroscopy ( Fig. 2a,b ). Compared with the free ligand, the peak of H e on benzimidazole of the assembly was shifted downfield from 8.77 to 9.00 p.p.m., suggesting the loss of electron density on the imidazole ring due to coordination or the involvement of Hydrogen bonding. The diastereotopic environment of the methylene protons, which split into a pair of doublets in a 1:1 ratio, indicates a cis conformation of the ligands in the product [44] . Diffusion-ordered NMR spectrum (DOSY) ( Supplementary Fig. 4 ) confirmed that all peaks have the same diffusion coefficient, with an estimated diameter of 1.12 nm for the assembly. The composition of product formulated as Pd 3 L 6 (NO 3 ) 6 ( 2 ) was then clearly provided by high-resolution ESI-TOF-MS. Prominent peaks observed at m/z =1028.1468, and 665.1049 correspond to the multiple-charged [ 2 –(NO 3 − ) n ] n + ( n =2, 3) molecular-ion signals, with consecutive loss of the NO 3 − counter-ions. Moreover, the isotopic patterns of each resolved peaks were also in good agreement with the simulated values ( Fig. 2g ). 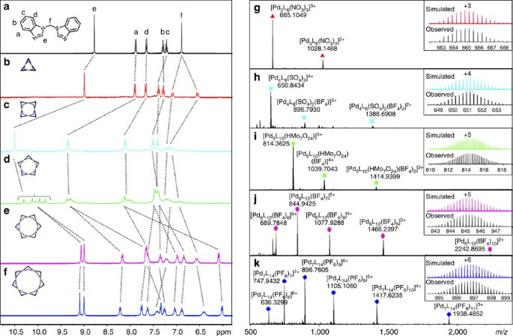Figure 2:1H NMR and ESI-TOF-MS spectra. (a–f) are1H NMR (400 MHz, [D6]DMSO, 298 K) spectra for free ligand1and the complexes2,3,4,5,6, respectively; (g–k) are ESI-TOF-MS spectra for complexes2,3,4,5and6with insets showing the representative observed and calculated isotope patterns. Figure 2: 1 H NMR and ESI-TOF-MS spectra. ( a – f ) are 1 H NMR (400 MHz, [D 6 ]DMSO, 298 K) spectra for free ligand 1 and the complexes 2 , 3 , 4 , 5 , 6 , respectively; ( g – k ) are ESI-TOF-MS spectra for complexes 2 , 3 , 4 , 5 and 6 with insets showing the representative observed and calculated isotope patterns. Full size image To our surprise, a clearly distinct product was obtained when Pd(BF 4 ) 2 was used during the self-assembly, in a similar reaction condition as described above (See Methods section for details). As shown in Fig. 2e , all the proton signals of the ligand on this complex strongly split into two sets in a 1:1 ratio, with one set of signals obviously downfield shifted and the other upfield shifted (except for the CH on imidazole) with respect to those of the free ligand. Such observation is clearly different from the trinuclear compound 2 , where only the protons on the methylene groups are split. This suggests two different chemical environments for the benzoimidazole moities in the final product. On the basis of 1 H- 1 H COSY experiment, all the signals could be fully assigned ( Supplementary Fig. 8 ). DOSY spectrum ( Supplementary Fig. 9 ) reveals the formation of a new product with an estimated diameter of 2.23 nm, which is dramatically larger than that of 2 . ESI-TOF-MS ( Fig. 2j ) discloses that this complex is formulated as Pd 6 L 12 ·(BF 4 ) 12 ( 5 ), with prominent peaks observed at m/z =689.7848, 844.9425, 1077.9288, 1466.2397 and 2242.8695, corresponding to [ 5 –(BF 4 − ) n ] n + ( n =2–6). On the basis of this unexpected structural switch from Pd 3 L 6 to Pd 6 L 12 by varing the counter ions from NO 3 − to BF 4 − , we then postulate that other counter ions with larger size may induce the formation of higher nuclear assembly. Indeed, pure heptanuclear Pd 7 L 14 ·(PF 6 ) 14 ( 6a ) or Pd 7 L 14 (OTf) 14 ( 6b ) complexes were quantitatively obtained by replacing the metal source with Pd(PF 6 ) 2 or Pd(OTf) 2 , respectively, the composition of which were determined in a similar manner by NMR and ESI-TOF-MS ( Fig. 2f,k and Supplementary Figs 13–21 ). Similar diastereotopic splitting of 1 H NMR signals into 1:1 ratio was also observed for compound 6 . Direct synthesis of the missing Pd n L 2 n macrocycles between n =3 and 6 were unsuccessful. Instead, the intermediate-sized Pd 4 L 8 and Pd 5 L 10 could be obtained by anion-induced transformation processes. In a typical procedure, tetrabutylammonium hydrogen sulfate (10.27 mg, 30.24 μmol, 4.5 eq.) was added to a 1 ml [D 6 ]DMSO solution of compound 5 (6.72 μmol) and the mixture was heat at 70 °C for 3 h. 1D ( Fig. 2c ) and 2D NMR ( Supplementary Figs 25 and 26 ) indicated the total transformation of 5 into a new product. In the 1 H NMR, the diagnostic diastereomeric splitting of the ligands signals on 5 gradually disappeared with the origin of another single set of signals (except for the methylene protons). Moreover, H e on the imidazole rings were significantly shifted downfield from 8.75 p.p.m. and 7.86 p.p.m. to 10.46 p.p.m. ), indicating the involvement of strong Hydrogen-bonding interactions with the bisulfate ions. DOSY revealed that the new complex was of a diameter of 1.51 nm, a value in between of the compound 2 and 5 . Even with intrinsic mixed counter anions, ESI-TOF-MS spectrum clearly confirmed the formation of the tetranuclear Pd 4 L 8 compound ( 3 ), with prominent peaks observed at m/z =650.8434, 896.7930, 1388.6908, corrsponding to [Pd 4 L 8 (SO 4 ) 2 ] 4+ , [Pd 4 L 8 (SO 4 ) 2 (BF 4 ) 1 ] 3+ , [Pd 4 L 8 (SO 4 ) 2 (BF 4 ) 2 ] 2+ , respectively. The loss of protons on bisulfates anions was possibly due to the total 8+ charge on the host or the presence of multiple Hydrogen bonding between the host and anions. Under similar conditions, induced-fit transformation from 6 to 3 was also quantitative (see discussion below). The conversion from M 6 L 12 to the M 5 L 10 structure was beyond anticipation. Our initial thought was to induce the formation of higher-nuclear Pd n L 2 n complexes (for n >7), using bulkier counter-ions. However, treating compound 5 (6.72 μmol) with 0.8 eq. tetrabutylammonium heptamolybdate (( t -Bu 4 N) 6 Mo 7 O 24 , 13.48 mg, 5.38 μmol) in 1 ml [D 6 ]DMSO solution converted 5 into Pd 5 L 10 ( 4 ) (same conditions as above). The formation of this new complex was indicated by 1 H NMR ( Fig. 2d ), where all signals become severely broadened with the H e significantly split into a complicated pattern, presumably due to a mismatch of symmetry between the host and the guest anion. However, 1 H NMR at 100 °C becomes much simplified ( Supplementary Fig. 30 ). In particular, the complicated pattern observed for H e coalesced into one single broadened peak with clear upfield-shifting, indicating the break of H bonds and increase of symmetry at elevated temperatures. DOSY revealed that the new complex was of a diameter of 1.84 nm ( Supplementary Fig. 34 ). ESI-TOF-MS reveals that a new pentanuclear Pd 5 L 10 compound ( 4 ) with an encapsulated [HMo 7 O 24 ] 5− cluster was formed, with prominent peaks observed at m/z = 814.3625, 1039.7043 and 1414.9399 corresponding to [Pd 5 L 10 (HMo 7 O 24 ) 1 ] 5+ , [Pd 5 L 10 (HMo 7 O 24 ) 1 (BF 4 ) 1 ] 4+ and [Pd 5 L 10 (HMo 7 O 24 )(BF 4 ) 2 ] 3+ , respectively ( Fig. 2i ). The structures of the self-assembled Pd n L 2 n complexes for n =3, 4, 5, 6 were unambiguously determined by single crystal diffraction studies facilitated by high-power X-ray source at the Shanghai Synchrotron Radiation Facility (SSRF). Crystal structures reveal that all complexes shares a similar donut-shaped structure, where 2n bent bidentate ligands are connected by n square-planar coordinated Pd II ions in a cyclic fashion. Ligands can be divided into two layers by an imaginary plane of the metal centres. On the basis of crystal structures, we can clearly see that hydrogen-bonding interactions between the host framework and its entrapped anions played an important role in dictating the size of the macrocycles. High quality single crystals of compound 2 suitable for crystallographic analysis were obtained by slow vapour diffusion of dichloromethane (DCM) into a DMSO solution of the complex over 3 weeks, which crystallized in a P –1 space group with two macrocycles sitting in the unit cell. This smallest donut-shaped assembly has an out diameter of 1.74 nm and a height of 0.87 nm, which can be regarded as a trimeric structure consisting three Pd 2 L 2 square building blocks by sharing the Pd II centres ( Fig. 3a,b ). Interestingly, three nitrate anions were H bonded inside the cavity, which form a three-layered sandwich conformation. One NO 3 − is in a perpendicular orientation to the other two parallel ones, possibly due to electrostatic repulsion. Each nitrate is involved in at least six Hydrogen-bonding interactions with the inward CH from the imidazole and methylene groups. We propose these multi-point H bonds act as glues to tie the ligand strands together. Similarly, diffusion of DCM into a DMSO solution of 3 resulted in the crystalization of this tetranuclear species ( Fig. 3c,d ). Two SO 4 2− are encapsulated inside the cavity in this case, each of which is sextuple H bonded with three ligands on the same layer. 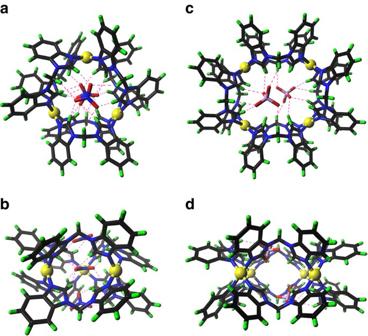Figure 3: X-ray single crystal structures of compounds 2 and 3. Top (a,c) and side (b,d) views of the X-ray crystal structures of compounds2and3. (Colour scheme: H bondings, red dashed lines; Pd, yellow; C, black; N, blue; S, pink; O, red; H, green. Solvents and anions located outside the macrocycles are omitted for clarity.) Figure 3: X-ray single crystal structures of compounds 2 and 3. Top ( a , c ) and side ( b , d ) views of the X-ray crystal structures of compounds 2 and 3 . (Colour scheme: H bondings, red dashed lines; Pd, yellow; C, black; N, blue; S, pink; O, red; H, green. Solvents and anions located outside the macrocycles are omitted for clarity.) Full size image Crystals for the Pd 5 L 10 complex ( 4 ) were also obtained by a similar method described above. The pentagonal topology of the framework was clearly confirmed ( Fig. 4a,b ). Possibly due to the mismatch of symmetry in this host-guest complex, modelling of the encapsulated HMo 7 O 24 5− anion with the known connectivity [48] , [49] were unsuccessful and its contribution was removed by the SQUEEZE routine [50] . We propose that the HMo 7 O 24 5− guest inside the confined cavity is severely disordered or adopting an unusual geometry. It has to be pointed out that the nature of the encapsulated [HMo 7 O 24 ] 5− cluster is unclear at this stage and detailed host-guest chemistry of these macrocycles with polyoxometalates deserves further study. After a long trail-and-error, high quality single crystals of 5 were fortunately obtained by a co-crystallization method with 1.0 eq. of NaB(ArF) 4 (ArF=3,5-bis(trifluoromethyl)phenyl). At this condition, 1 H or 19 F NMR ( Supplementary Figs 10 and 11 ) did not show obvious chemical shift for both the host and the [B(ArF) 4 ] − anion, indicating that there is no strong interaction between them. Compound 5 crystallized in an orthogonal R –3c space group with a huge unite cell volume of 119,056 Å 3 ( Fig. 4c,d ). The dimension of this self-assembled macrocycle spans an out diameter of 2.24 nm and inner diameter of 1.19 nm. Compared to the symmetrical Pd 2 L 2 squares units existing on the crystal structures of 2 , 3 and 4 , the six Pd 2 L 2 units on 5 were severely distorted into a rectangular conformation, which provides a good reason for the split signals observed in its 1 H NMR. Such structural distortion also reflects the flexibility of ligand 1 . Due to the low-diffraction nature of this sample, only the Pd 6 L 12 connectivity was confirmed and no detailed anion binding mode could be modelled. In crystal packing, two giant channels are present along the c axis due to layer-by-layer stacking of the ring-shaped complexes, one of which is defined by the ring cavity with a diameter of 1.19 nm, the other is 1.75 nm encircled by six adjacent molecules, where we hypothesize is filled with the highly disordered bulky [B(ArF) 4 ] − anions. Many attempts to crystallize the heptanuclear 6 were unsuccessful, possibly due to its low symmetry and big size. This structure was then modelled by molecular mechanical optimizations and depicted in Fig. 4e,f . 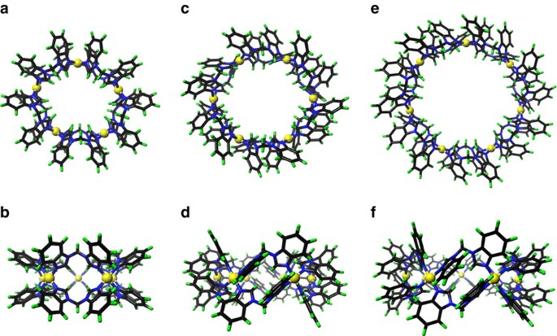Figure 4: X-ray single crystal structures of compounds 4, 5 and simulated structures of complex 6. Top (a,c) and side (b,d) views for the X-ray crystal structures of complexes4and5; (e,f) are similar views for the simulated structure of complex6. (Same colour schemes were used as forFig. 3.) Figure 4: X-ray single crystal structures of compounds 4, 5 and simulated structures of complex 6. Top ( a , c ) and side ( b , d ) views for the X-ray crystal structures of complexes 4 and 5 ; ( e , f ) are similar views for the simulated structure of complex 6 . (Same colour schemes were used as for Fig. 3 .) Full size image Taking advantage of the anion-adaptivity observed during the self-assembly, we then managed to draw a comprehensive map detailing the induced-fit transformation processes between all species of the family ( Fig. 5a and Supplementary Figs 42–58 ). First of all, we found that addition of 30 eq. of KNO 3 to the Pd 7 L 14 complex (PF 6 − salt) or Pd 6 L 12 complex 5 resulted in the quantitative transformation to Pd 3 L 6 . The (Mo 7 O 24 )@Pd 5 L 10 was found to be the the most stable host-guest complex for this dynamic combinatorial system, which could be quantitatively obtained by additon of ( t -Bu 4 N) 6 Mo 7 O 24 to either compounds 2 , 3 , 5 or 6 . In fact, this host-guest complex is so stable that once formed it will never transform into other macrocycles. Similarly, Pd 3 L 6 could be quantitatively obtained by the templation effect of the NO 3 − anion starting from Pd 4 L 8 , Pd 6 L 12 or Pd 7 L 14 . SO 4 2− , on the contrary, is a weaker template comparing to NO 3 − , possibly due to the fact that Pd 3 L 6 can encapsulate three NO 3 − while Pd 4 L 8 can only host two SO 4 2− . Meanwhile, transformation from Pd 7 L 14 to Pd 6 L 12 was obtained in only 80% yield even if 35 eq. of BF 4 − anion was used, suggesting only a subtle energy difference between them. On the basis of this map, a sequence of templating-effect like Mo 7 O 24 6− >NO 3 − >SO 4 2− >BF 4 − >PF 6 − =OTf − was obtained for this dynamic combinatorial system. 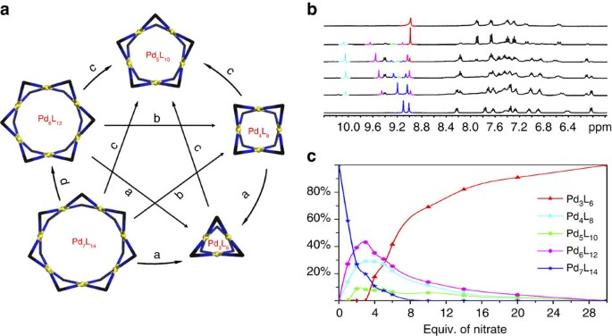Figure 5: Induce-fit transformations between macrocycles. (a) Cross map showing all the transformations between the macrocyclic species (conditions for a: NO3−; b: HSO4−; c: Mo7O246−; d: BF4−); (b)1H NMR (400 MHz, [D6]DMSO, 298 K) titration spectra showing the gradual transformation from the heptanuclear complex6ato the trinuclear complex2by sequential addition of KNO3(bottom up: 0, 1, 2, 4, 10, 30 eq.) with Hesignals highlighted for Pd3L6: red, Pd4L8: sky blue, Pd5L10: green, Pd6L12: pink and Pd7L14: dark blue, respectively; (c) Composition distributions for all the PdnL2nspecies obtained by the integrals of the Hesignals from the titration experiment. Figure 5: Induce-fit transformations between macrocycles. ( a ) Cross map showing all the transformations between the macrocyclic species (conditions for a: NO 3 − ; b: HSO 4 − ; c: Mo 7 O 24 6− ; d: BF 4 − ); ( b ) 1 H NMR (400 MHz, [D 6 ]DMSO, 298 K) titration spectra showing the gradual transformation from the heptanuclear complex 6a to the trinuclear complex 2 by sequential addition of KNO 3 (bottom up: 0, 1, 2, 4, 10, 30 eq.) with H e signals highlighted for Pd 3 L 6 : red, Pd 4 L 8 : sky blue, Pd 5 L 10 : green, Pd 6 L 12 : pink and Pd 7 L 14 : dark blue, respectively; ( c ) Composition distributions for all the Pd n L 2 n species obtained by the integrals of the H e signals from the titration experiment. Full size image Finally, a detailed tranformation process from Pd 7 L 14 ( 6a ) to Pd 3 L 6 was traced by titration experiments following the sequential addition of NO 3 − ( Fig. 5b,c ). 1 H NMR and ESI-TOF-MS showed that the transformation took place via a gradual shrinking of the macrocyclic framework. On the basis of a careful assignment of the NMR and ESI-TOF-MS signals ( Supplementary Figs 59–70 and Supplementary Tables 5 and 6 ), it was found that after adding 1 eq. of NO 3 − ([NO 3 − ]:[PF 6 − ]=1:14) the Pd 7 L 14 macrocycle starts to transform into Pd 6 L 12 and Pd 4 L 8 , whose contents reach maxima when 3 eq. of NO 3 − were added. Meanwhile, formation of Pd 5 L 10 was also detected starting from the addition of 2 eq. of NO 3 − . All of these intermediates start to drop in contents after the most stable Pd 3 L 6 complex evolved in the system. We hypothesize that NO 3 − anions are acting as hydrogon-bonding anchors which pull together the neighbouring Pd 2 L 2 square units on the framework, leading to a gradually shrinking of the ring size. The contents of Pd 6 L 12 and Pd 4 L 8 are aboundent during the transformation proecess, possibly due to the fact that they have even numbers of Pd 2 L 2 square units, which can maximize the number of H bonding with the NO 3 − anchors. In contrast, the concentration of the Pd 5 L 10 intermediate, which has odd number of Pd 2 L 2 square units, was rather low ( Supplementary Fig. 71 ). In summary, a dynamic anion-adaptive self-assembly system was constructed consisting of a very simple ligand and Pd II ions. The anion-induced transformation between the Pd n L 2 n species are reminiscent of the induced-fit guest-binding mechanism observed in nature. Moreover, this new class of donut-shaped assemblies provide unique tunable hydrogen-binding pockets, where we envisage molecular sensing/catalysis is possible to take place. Materials Unless otherwise noted, all chemicals and solvents were purchased from commercial corporations and used without further purification. Deuterated solvents were purchased from Admas and J&K scientific. NMR measurements 1D and 2D NMR spectra were measured on a Bruker-BioSpin AVANCE Ш HD (400 MHz) spectrometer. 1 H NMR chemical shifts were determined with respect to residual solvent signals of the deuterated solvents used. DOSY spectra were applied to estimate the dynamic radius for the compounds 2 , 3 , 4 , 5 and 6 according to the Stokes-Einstein equation (1). Where: D is diffusion coefficient obtained from DOSY spectrum, K B is Boltzmann constant, T is temperature, viscosity η was tested to be 2.2 mPa s and r is the estimated dynamic radius. MS measurements ESI-Q-TOF mass spectra were recorded on an Impact II UHR-TOF mass spectrometry from Bruker, with ESI-L low concentration tuning mix (from Agilent Technologies) as the internal standard (Accuracy <3 p.p.m.). Data analyses and simulations of ESI-TOF mass spectra were processed on a Bruker Data Analysis software (Version 4.3). Molecular mechanical structure simulations were performed on a Material Studio v6.0 software using the build-in geometry optimization task based on the Universal forcefield. Synthesis and characterization (Pd 3 L 6 )(NO 3 ) 6 (2) Ligand 1 (ref. 51 ) (4.98 mg, 20.07 μmol) was treated with Pd(NO 3 ) 2 (10.04 μmol) in [D 6 ]DMSO (1 ml) at 70 °C for 5 h. 1 H NMR confirmed the quantitative formation of complex 2 . 1 H NMR (400 MHz, [D 6 ]DMSO, 298 K) δ 8.99 (s, 12H), 7.90 (d, J =8.3 Hz, 12H), 7.66 (d, J =8.3 Hz, 12H), 7.39 (t, J =7.8 Hz, 12H), 7.28 (t, J =7.8 Hz, 12H), 7.09 (d, J =13.7 Hz, 6H), 6.55 (d, J =14.0 Hz, 6H). 13 C NMR (100 MHz, [D 6 ]DMSO, 298 K) δ 145.39, 138.88, 130.67, 125.99, 124.90, 117.77, 111.82 and 54.51( Supplementary Figs 1–3 ). ESI-TOF-MS (NO 3 − salt, CH 3 CN): the following picked signals are those at the highest intensities. m/z Calcd for [Pd 3 L 6 (NO 3 − ) 4 ] 2+ 1028.1513, found 1028.1468; Calcd for [Pd 3 L 6 (NO 3 − ) 3 ] 3+ 665.1049, found 665.1049 ( Supplementary Fig. 5 ). (Pd 6 L 12 )(BF 4 ) 12 (5) PdCl 2 (17.73 mg, 0.10 mmol) was dissolved in [D 6 ]DMSO (2 ml) and stirred for 10 h at room temperature with AgBF 4 (38.94 mg, 0.20 mmol). After removal of AgCl by filtration, the Pd(BF 4 ) 2 stock solution in [D 6 ]DMSO was obtained quantitatively. Ligand 1 (20.00 mg, 80.60 μmol) was treated with Pd(BF 4 ) 2 (40.30 μmol) in [D 6 ]DMSO (1 ml) at 70 °C for 5 h. After addition of 0.3 ml DCM into the solution, a small amount of precipitation appeared which was then filtrated off and pure compound 5 in [D 6 ]DMSO was obtained after removal of DCM. The isolation yield of this compound is about 65%. 1 H NMR (400 MHz, [D 6 ]DMSO, 298 K) δ 9.06 (s, 12H), 9.00 (s, 12H), 8.17 (d, J =8.2 Hz, 12H), 7.63 (dd, J =17.0, 8.0 Hz, 36H), 7.35 (t, J =7.8 Hz, 12H), 7.22 (d, J =14.6 Hz, 12H), 6.99 (t, J =7.8 Hz, 12H), 6.84 (t, J =7.5 Hz, 12H), 6.57 (d, J =14.8 Hz, 12H), 6.09 (d, J =8.2 Hz, 12H). 19 F NMR (376 MHz, [D 6 ]DMSO, 298 K) δ -147.31. 13 C NMR (100 MHz, [D 6 ]DMSO, 298 K) δ 146.12, 144.82, 138.32, 138.20, 132.34, 128.63, 126.92, 126.53, 126.02, 125.64, 117.88, 117.39, 111.96, 110.55 and 54.36 ( Supplementary Figs 6–11 ). ESI-TOF-MS (BF 4 − salt, CH 3 CN): the following picked signals are those at the highest intensities. m/z Calcd for [(Pd 6 L 12 )(BF 4 ) 9 ] 3+ 1466.2455, found 1466.2397; Calcd for [(Pd 6 L 12 )(BF 4 ) 8 ] 4+ 1077.9331, found 1077.9288; Calcd for [(Pd 6 L 12 )(BF 4 ) 7 ] 5+ 844.9456, found 844.9425; Calcd for [(Pd 6 L 12 )(BF 4 ) 6 ] 6+ 689.7873, found 689.7848 ( Supplementary Fig. 12 ). (Pd 7 L 14 )(PF 6 ) 14 (6a) PdCl 2 (17.73 mg, 0.10 mmol) was dissolved in DMSO (2 ml) and stirred for 10 h at room temperature in dark with AgPF 6 (50.57 mg, 0.20 mmol). After removal of AgCl by filtration, stock solution of Pd(PF 6 ) 2 in [D 6 ]DMSO was obtained quantitatively. Then ligand 1 (20 mg, 80.60 μmol) was treated with Pd(PF 6 ) 2 (40.30 μmol) in [D 6 ]DMSO (1 ml) at 70 °C for 5 h. 1 H NMR confirmed the quantitative formation of complex. 1 H NMR confirmed the quantitative formation of complex 6a . 1 H NMR (400 MHz, [D 6 ]DMSO, 298 K) δ 9.09 (s, 14H), 9.00 (s, 14H), 8.22 (d, J =8.4 Hz, 14H), 7.76 (d, J =8.2 Hz, 14H), 7.63 (t, J =7.5 Hz, 14H), 7.42 (d, J =12.7 Hz, 14H), 7.35 (d, J =8.4 Hz, 14H), 7.30–7.22 (m, 14H), 7.04 (t, J =7.6 Hz, 14H), 6.89 (t, J =7.6 Hz, 14H), 6.41 (d, J =13.7 Hz, 14H), 6.02 (d, J =8.2 Hz, 14H). 13 C NMR (100 MHz, [D 6 ]DMSO, 298 K) δ 145.32, 144.72, 138.06, 137.49, 132.14, 128.38, 126.81, 125.89, 117.40, 116.90, 111.79, 110.31 and 54.16 ( Supplementary Figs 13–15 ). ESI-TOF-MS (PF 6 − salt, CH 3 CN): the following picked signals are those at the highest intensities. m/z Calcd for [(Pd 7 L 14 )(PF 6 ) 11 ] 3+ 1938.4758, found 1938.4852; Calcd for [(Pd 7 L 14 )(PF 6 ) 10 ] 4+ 1417.6157, found 1417.6235; Calcd for [(Pd 7 L 14 )(PF 6 ) 9 ] 5+ 1105.0996, found 1105.1060; Calcd for [(Pd 7 L 14 )(PF 6 ) 8 ] 6+ 896.7555, found 896.7605; Calcd for [(Pd 7 L 14 )(PF 6 ) 7 ] 7+ 747.9384, found 747.9432; Calcd for [(Pd 7 L 14 )(PF 6 ) 6 ] 8+ 636.3255, found 636.3299 ( Supplementary Fig. 20 ). (Pd 7 L 14 )(CF 3 SO 3 ) 14 (6b) PdCl 2 (17.73 mg, 0.10 mmol) was dissolved in [D 6 ]DMSO (2 ml) and stirred for 10 h at room temperature in dark with AgCF 3 SO 3 (51.39 mg, 0.20 mmol). After removal of AgCl by filtration, the stock solution of Pd(CF 3 SO 3 ) 2 in [D 6 ]DMSO was obtained quantitatively. Then ligand 1 (10 mg, 40.29 μmol) was treated with Pd(CF 3 SO 3 ) 2 (20.15 μmol) in [D 6 ]DMSO (1 ml) at 70 °C for 5 h. 1 H NMR confirmed the quantitative formation of complex 6b . 1 H NMR (400 MHz, [D 6 ]DMSO, 298 K) δ 9.19 (d, J =8.6 Hz, 28H), 8.21 (d, J =8.2 Hz, 14H), 7.72 (d, J =7.9 Hz, 14H), 7.65–7.55 (m, 14H), 7.40–7.28 (m, 28H), 7.27–7.17 (m, 14H), 7.07–6.96 (m, 14H), 6.91–6.80 (m, 14H), 6.53 (d, J =14.5 Hz, 14H), 6.00 (d, J =7.8 Hz, 14H). 13 C NMR (100 MHz, [D 6 ]DMSO, 298 K) δ 145.32, 144.72, 138.06, 137.49, 132.14, 128.38, 126.81, 125.89, 117.40, 116.90, 111.79, 110.31 and 54.16 ( Supplementary Figs 16–18 ). ESI-TOF-MS (CF 3 SO 3 − salt, CH 3 CN): the following picked signals are those at the highest intensities. m/z Calcd for [(Pd 7 L 14 )(CF 3 SO 3 ) 11 ] 3+ 1953.4308, found 1953.4414; Calcd for [(Pd 7 L 14 )(CF 3 SO 3 ) 10 ] 4+ 1427.8350, found 1427.8426; Calcd for [(Pd 7 L 14 )(CF 3 SO 3 ) 9 ] 5+ 1112.4775, found 1112.4827; Calcd for [(Pd 7 L 14 )(CF 3 SO 3 ) 8 ] 6+ 902.2392, found 902.2435; Calcd for [(Pd 7 L 14 )(CF 3 SO 3 ) 7 ] 7+ 751.9261, found 751.9297; Calcd for [(Pd 7 L 14 )(CF 3 SO 3 ) 6 ] 8+ 751.9261, found 751.9297; Calcd for [(Pd 7 L 14 )(CF 3 SO 3 ) 5 ] 9+ 639.3163, found 639.3199 ( Supplementary Fig. 21 ). (Pd 4 L 8 )(SO 4 ) 2 (BF 4 ) 4 (3) the solution of 5 (6.72 μmol) was treated with tetrabutylammonium hydrogen sulfate (10.27 mg, 30.24 μmol, 4.50 eq.) at 70 °C for 3 h. 1 H NMR confirmed the quantitative formation of complex 3 . 1 H NMR (400 MHz, [D 6 ]DMSO, 298 K) δ 10.46 (s, 16H), 9.30 (d, J =8.4 Hz, 16H), 8.06 (d, J =8.5 Hz, 16H), 7.46 (t, J =7.7 Hz, 16H), 7.36 (t, J =7.6 Hz, 16H), 7.16 (d, J =15.4 Hz, 8H), 7.07 (d, J =14.8 Hz, 8H). 13 C NMR (100 MHz, DMSO, 298 K) δ 145.61, 138.53, 132.16, 125.77, 124.92, 118.68, 112.05 and 57.76 ( Supplementary Figs 22–25 ). ESI-TOF-MS (SO 4 2− /BF 4 − salt, CH 3 CN): the following picked signals are those at the highest intensities. m/z Calcd for [(Pd 4 L 8 )(SO 4 ) 2 (BF 4 ) 2 ] 2+ 1388.6898, found 1388.6908; Calcd for [(Pd 4 L 8 )(SO 4 ) 2 (BF 4 )] 3+ 896.7918, found 896.7930; Calcd for [(Pd 4 L 8 )(SO 4 ) 2 ] 4+ 650.8428, found 650.8434 ( Supplementary Figs 27 and 28 ). (Pd 5 L 10 )(HMo 7 O 24 )(BF 4 ) 5 (4) the solution of 5 (6.72 μmol) was treated with tetrabutylammonium heptamolybdate (13.48 mg, 5.38 μmol, 0.80 eq.) at 70 °C for 3 h. 1 H NMR confirmed the quantitative formation of complex 4 . 1 H NMR (400 MHz, [D 6 ]DMSO, 298 K) δ 10.01 (ddd, J =65.3, 61.9, 39.5 Hz, 20H), 9.28 (t, J =28.2 Hz, 20H), 8.21–7.91 (m, 20H), 7.42 (d, J =8.0 Hz, 20H), 7.37 (s, 20H), 7.18 (s, 10H), 6.91 (s, 10H). 13 C NMR (100 MHz, DMSO,298 K) δ 144.61, 138.26, 130.82, 125.10, 124.49, 119.10 and 111.60 ( Supplementary Figs 29–33 ). ESI-TOF-MS (HMo 7 O 24 5− , BF 4 − salt, CH 3 CN): the following picked signals are those at the highest intensities. m/z Calcd for [(Pd 5 L 10 )(HMo 7 O 24 )] 5+ 814.3625, found 814.3622; Calcd for [(Pd 5 L 10 )(HMo 7 O 24 )(BF 4 )] 4+ 1039.7043, found 1039.7051; Calcd for [(Pd 5 L 10 )(HMo 7 O 24 )(BF 4 ) 2 ] 3+ 1414.9399, found 1414.9400 ( Supplementary Figs 35 and 36 ). Transformation of 6a into 5 by BF 4 − : 35 eq. of N(C 4 H 9 ) 4 BF 4 was added into the prepared solution of compound 6a, followed by stirring for 3 h at 70 °C. 1 H NMR and ESI-TOF-MS spectra revealed that compound 6a changed into 5 (with mixed counter anions of PF 6 − and BF 4 − ) in 80% yield ( Supplementary Figs 42–44 and Supplementary Table 5 ). Transformation of 6a into 4 by Mo 7 O 24 6− : 0.8 eq. of [N(C 4 H 9 ) 4 ] 6 Mo 7 O 24 was added into the prepared solution of compound 6a, followed by stirring for 3 h at 70 °C. 1 H NMR and ESI-TOF-MS spectra revealed that compound 6a quantitatively changed into 4 (with mixed counter anions of PF 6 − and HMo 7 O 24 5− ) ( Supplementary Figs 36 and 45 ). Transformation of 6a into 3 by HSO 4 − : 5.25 eq. of N(C 4 H 9 ) 4 HSO 4 was added into the prepared solution of compound 6a, followed by stirring for 3 h at 70 °C. The 1 H NMR and ESI-TOF-MS spectra revealed that the compound 6a quantitatively changed into 3 (with mixed counter anions of PF 6 − and SO 4 − ) completely ( Supplementary Figs 28 and 46 ). Transformation of 6a into 2 by NO 3 − : 30 eq. of KNO 3 was added into the prepared solution of compound 6a, followed by stirring for 3 h at 70 °C. The 1 H NMR and ESI-TOF-MS spectra revealed the compound 6a quantitatively changed into 2 (with mixed counter anions of PF 6 − and NO 3 − ) completely ( Supplementary Figs 47 and 48 ). Transformation of 5 into 4 by Mo 7 O 24 6− : 0.8 eq. of [N(C 4 H 9 ) 4 ] 6 Mo 7 O 24 was added into the prepared solution of compound 5, followed by stirring for 3 h at 70 °C. The 1 H NMR and ESI-TOF-MS spectra revealed that compound 5 quantitatively changed into 4 (with mixed counter anions of BF 4 − and HMo 7 O 24 5− ) ( Supplementary Figs 49–35 ). Transformation of 5 into 3 by HSO 4 − : 4.5 eq. of N(C 4 H 9 ) 4 HSO 4 was added into the prepared solution of compound 5, followed by stirring for 3 h at 70 °C. The 1 H NMR and ESI-TOF-MS spectra revealed the compound 5 quantitatively changed into 3 (with mixed counter anions of BF 4 − and SO 4 − ) ( Supplementary Figs 27 and 50 ). Transformation of 5 into 2 by NO 3 − : 12 eq. of KNO 3 was added into the prepared solution of compound 5, followed by stirring for 3 h at 70 °C. The 1 H NMR and ESI-TOF-MS spectra revealed the compound 5 quantitatively changed into 2 (with mixed counter anions of BF 4 − and NO 3 − ) ( Supplementary Figs 51 and 52 ). Transformation of 3 into 4 by Mo 7 O 24 6− : 2.4 eq. of [N(C 4 H 9 ) 4 ] 6 Mo 7 O 24 was added into the prepared solution of compound 3, followed by stirring for 3 h at 70 °C. The 1 H NMR and ESI-TOF-MS spectra revealed the compound 3 quantitatively changed into 4 (with mixed counter anions of HSO 4 − , BF 4 − and HMo 7 O 24 5− ) ( Supplementary Figs 53 and 54 ). Transformation of 3 into 2 by NO 3 − : 13.3 eq. of KNO 3 was added into the prepared solution of compound 3, followed by stirring for 3 h at 70 °C. The 1 H NMR and ESI-TOF-MS spectra revealed the compound 3 quantitatively changed into 2 (with mixed counter anions of HSO 4 − , BF 4 − and NO 3 − ) ( Supplementary Figs 56 and 55 ). Transformation of 2 into 4 by Mo 7 O 24 6− : 2 eq. of [N(C 4 H 9 ) 4 ] 6 Mo 7 O 24 was added into the prepared solution of compound 2, followed by stirring for 3 h at 70 °C. The 1 H NMR and ESI-TOF-MS spectra revealed that compound 2 quantitatively changed into 4 (with mixed counter anions of NO 3 − and HMo 7 O 24 5− ) ( Supplementary Figs 57 and 58 ). Single crystal X-ray diffractions The X-ray diffraction studies for complexes 2 , 3 , 4 , 5 were carried out at the BL17B macromolecular crystallography beamline in SSRF. The collected diffraction data were processed with the HKL2000 software program [52] . All the structures were solved by direct methods and refined by full-matrix least-squares on F 2 with anisotropic displacement using the SHELX software package [53] . The crystals of these kinds of giant supramolecular assemblies often diffract very weekly in nature. Some of the final R factors were converged to very high values, because the crystal was diffracting very weakly due to a large amount of disordered/amorphous solvents and anions that could not be fully located. The electron residuals in such cases were removed by the SQUEEZE routine [54] . We tried our best to finish the refinement but still some A-alerts are found by the (IUCr) checkCIF routine, all of which are due to the poor diffraction nature of the crystals or the disorder of the solvents and anions. Details on crystal data collection and refinement were summarized in Supplementary Tables 1–4 . Crystal data for 2 : space group P-1 , a =18.088(4) Å, b =18.299(4) Å, c =20.871(4) Å, V =6,099(3) Å 3 , Z =2, T =80 K. Anisotropic least-squares refinement for the framework atoms and isotropic refinement for the other atoms on 30,186 independent merged reflections ( R int =0.0292) converged at residual wR 2 =0.3805 for all data; residual R 1 =0.1126 for 59494 observed data [ I >2 σ ( I )], and goodness of fit (GOF)=1.048. Crystal data for 3 : space group P21c , a =18.178(4) Å, b =32.042(6) Å, c =18.582(4) Å, V =10,616(4) Å 3 , Z =2, T =293 K. Anisotropic least-squares refinement for the framework atoms and isotropic refinement for the other atoms on 26,904 independent merged reflections ( R int =0.0809) converged at residual wR 2 =0.2780 for all data; residual R 1 =0.0765 for 93,650 observed data [ I >2 σ ( I )], and goodness of fit (GOF)=1.042. Crystal data for 4 : space group Pmmn , a= 20.3994(4) Å, b =21.2991(4) Å, c =29.5319(6) Å, V =12,831.3(4) Å 3 , Z =2, T =293 K. Anisotropic least-squares refinement for the framework atoms and isotropic refinement for the other atoms on 13,683 independent merged reflections ( R int =0.0591) converged at residual wR 2 =0.5449 for all data; residual R 1 =0.1540 for 18,8179 observed data [ I >2 σ ( I )], and goodness of fit (GOF)=2.991. Crystal data for 5 : space group R-3c , a =71.246(4) Å, b=71.246(4) Å, c=27.0831(16) Å, V= 119056(15) Å 3 , Z =18, T =293 K. Anisotropic least-squares refinement for the framework atoms and isotropic refinement for the other atoms on 10,282 independent merged reflections ( R int =0.145) converged at residual wR 2 =0.4507 for all data; residual R 1 =0.1369 for 96,189 observed data [ I >2 σ ( I )], and goodness of fit (GOF)=2.044. Data availability The X-ray crystallographic coordinates for structures reported in this article have been deposited at the Cambridge Crystallographic Data Centre (CCDC), under deposition nos CCDC 1529252-1529255. These data can be obtained free of charge ( http://www.ccdc.cam.ac.uk/data_request/cif ). All other data are either provided in the Article and its Supplementary Information or are available on request. How to cite this article: Zhang, T. et al . Adaptive self-assembly and induced-fit transformations of anion-binding metal-organic macrocycles. Nat. Commun. 8 , 15898 doi: 10.1038/ncomms15898 (2017). Publisher’s note: Springer Nature remains neutral with regard to jurisdictional claims in published maps and institutional affiliations.